Cholesterol selectively activates canonical Wnt signalling over non-canonical Wnt signalling Wnt proteins control diverse biological processes through β-catenin-dependent canonical signalling and β-catenin-independent non-canonical signalling. The mechanisms by which these signalling pathways are differentially triggered and controlled are not fully understood. Dishevelled (Dvl) is a scaffold protein that serves as the branch point of these pathways. Here, we show that cholesterol selectively activates canonical Wnt signalling over non-canonical signalling under physiological conditions by specifically facilitating the membrane recruitment of the PDZ domain of Dvl and its interaction with other proteins. Single-molecule imaging analysis shows that cholesterol is enriched around the Wnt-activated Frizzled and low-density lipoprotein receptor-related protein 5/6 receptors and plays an essential role for Dvl-mediated formation and maintenance of the canonical Wnt signalling complex. Collectively, our results suggest a new regulatory role of cholesterol in Wnt signalling and a potential link between cellular cholesterol levels and the balance between canonical and non-canonical Wnt signalling activities. Signalling by the Wnt family of glycolipoproteins plays a crucial role in cell proliferation, cell polarity and cell fate determination during embryonic development and tissue homeostasis [1] , [2] , [3] , [4] . Mutations or deregulated expression of Wnt signalling components are often linked to human birth defects, cancer and other diseases [1] , [2] , [3] , [4] . Dishevelled (Dvl/Dsh) (≈750 amino acids) is a scaffold protein that plays central and pleiotropic roles in Wnt signalling [5] . Three Dvl homologues (Dvl1–3) with high sequence homology and redundant activities have been identified in mammals [5] . In canonical Wnt signalling, Wnt ligands bind cell-surface receptors Frizzled (Fz) and low-density lipoprotein receptor-related protein 5/6 (LRP5/6), which results in recruitment of Dvl and Axin to the Fz–Wnt–LRP5/6 complex. This causes disassembly of the β-catenin destruction complex by a yet unknown mechanism [6] , leading to the nuclear accumulation of β-catenin and activation of the transcription of Wnt target genes. Dvl also mediates various β-catenin-independent, non-canonical Wnt signalling pathways, including the Rho/JNK-mediated planar cell polarity (PCP) pathway that controls actin cytoskeleton [7] . Owing to its critical involvement in cancer and other diseases, the canonical Wnt pathway has been a major target for drug development [8] , [9] , [10] , [11] , [12] . More recently, Dvl has emerged as an attractive target for therapeutic intervention [13] , [14] . Consistent with its complex functions, Dvl can interact with a wide range of protein partners involved in Wnt signalling using several conserved motifs and domains. The N-terminal DIX ( DI shevelled/A X in) domain mediates Dvl self-association [15] , which is important for LRP6 phosphorylation and propagation of canonical Wnt signalling [16] . The central PDZ ( P SD-95, D LG, Z O-1) domain is mainly involved in interaction with the activated Fz receptor [17] . The C-terminal DEP ( D vl, E GL-10, P leckstrin) domain has been reported to bind anionic lipids in the plasma membrane (PM) [18] and other proteins, including the intracellular loops of Fz5 (ref. 19 ). However, the mechanisms by which Dvl is recruited to the PM and interacts with ≈80 protein partners in a spatiotemporally specific manner, during diverse Wnt signalling pathways, are not fully understood. Furthermore, it is unknown how Dvl serves as a branch point for canonical and non-canonical Wnt signalling pathways. This complexity has hampered the development of potent and specific modulators of Dvl-mediated canonical Wnt signalling. Cholesterol is a major lipid component (that is, 30–40%) of the mammalian PM. While much is known about the metabolism and transport of cholesterol and its role in various human diseases [20] , less is known about the exact cellular function of cholesterol. Cholesterol has been implicated in regulation of physical properties of PM, formation of cholesterol-rich membrane microdomains [21] and structural and functional modulation of integral membrane proteins [22] . A recent proteomics study identified a large number of (that is, >250) cholesterol-binding proteins, suggesting a potential link between cellular cholesterol concentrations and diverse cellular processes [23] . However, the direct involvement of cholesterol in cell regulation through specific interactions with cellular proteins has not been thoroughly investigated. In this report, we show that cholesterol specifically interacts with the PDZ domain of Dvl (Dvl-PDZ) and facilitates the interaction of Dvl with key protein components of canonical Wnt signalling, leading to selective activation of the canonical Wnt signalling pathway over non-canonical Wnt signalling pathways. Dvl-PDZ domain specifically binds cholesterol To fully understand the mechanisms by which Dvl is recruited to the PM and differentially mediates canonical and non-canonical Wnt signalling, we focused on the biophysical characterization of the PDZ domain that plays a central role in Fz binding in both canonical and non-canonical Wnt signalling [5] , [24] . Although the main function of Dvl-PDZ in Wnt signalling is to interact with the activated Fz receptor [17] , the Dvl-PDZ–Fz interaction has been reported to be relatively weak [17] , [19] and nonspecific [13] . We therefore searched for a secondary interaction that may specifically drive the canonical Wnt signalling activity of Dvl-PDZ. It has been reported that many PDZ domains can effectively interact with membrane lipids [25] , [26] , [27] , [28] . To explore the possibility that lipid binding may specifically regulate the canonical Wnt signalling activity of Dvl-PDZ, we measured the binding of the PDZ domains of three Dvl proteins (that is, Dvl1–3) to vesicles whose lipid composition recapitulates that of the cytofacial leaflet of PM, where the Dvl-PDZ–Fz interaction takes place. 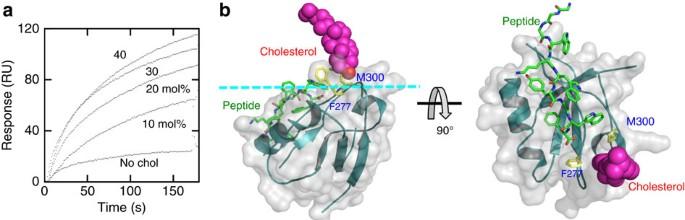Figure 1: Cholesterol binding of Dvl2-PDZ domain. (a) Cholesterol dependence of membrane binding of Dvl2-PDZ. Binding of the PDZ domain to POPC/POPS/cholesterol (80−x:20:x,x=0–40 mol%) vesicles was measured by SPR analysis. Notice that Dvl2-PDZ has significant binding to POPC/POPS (80:20) vesicles and thus the net affinity for cholesterol should be estimated by subtracting the sensorgram for POPC/POPS (80:20) vesicles from that of particular vesicles. Equilibrium SPR measurements were performed in 20 mM Tris-HCl, pH 7.4, containing 0.16 M KCl. POPC vesicles to which Dvl2-PDZ has no detectable affinity were used for the control surface. (b) A model structure of the Dvl2-PDZ–cholesterol–peptide ternary complex was obtained by docking cholesterol and the C-terminal Fz7 peptide to Dvl2-PDZ (PDB ID: 2REY). Cholesterol (with its hydrophobic tail pointing upwards) and the bound peptide are shown in space-filling and stick representations, respectively. Putative cholesterol-binding residues, F227 and M300, are shown in stick representation and labelled. They are predicted to partially penetrate the membrane and make contact with the hydrophobic A and B rings of cholesterol. The structure on the left panel is shown in a putative membrane-binding orientation with the dotted line indicating the membrane surface. The same model structure is also shown in a different orientation with the top surface facing the membrane (right panel). Notice that the putative lipid-binding sites are topologically distinct from the peptide-binding pocket. The model was built in the absence of the lipid bilayer and the protein may undergo further conformational changes when it binds the membrane. Surface plasmon resonance (SPR) analysis showed that they indeed have high affinity (that is, K d =30–50 nM) for the PM-mimetic vesicles (see Table 1 ; Supplementary Fig. 1 ). Among the three Dvl homologues, Dvl2 is the most conserved in all species [5] , [24] , and we thus further characterized Dvl2 and its PDZ domain (Dvl2-PDZ). To determine whether Dvl2-PDZ has selectivity for any lipid component of the PM-mimetic vesicles, we measured the effect of removing major lipid components, phosphatidylserine (PS) and cholesterol, and a key regulatory lipid, phosphatidylinositol-4,5-bisphosphate (PtdIns(4,5)P 2 ) [29] , [30] , from the PM-mimetic vesicles on its membrane affinity. When either PS or PtdIns(4,5)P 2 was deleted from the vesicles, Dvl2-PDZ had considerably weaker binding, indicating its dependence on anionic lipids for membrane binding ( Supplementary Fig. 2A ). Interestingly, removal of cholesterol from the PM-mimetic vesicles had the largest effect on the vesicle binding of Dvl2-PDZ ( Supplementary Fig. 2A ). Many cytosolic proteins and domains, including the DEP domain of Dvl (ref. 18 ), are known to be recruited to the PM by binding to anionic lipids [31] , [32] , [33] ; however, cholesterol-binding cytosolic proteins are rare [28] . We thus further investigated the cholesterol binding of Dvl2-PDZ. Dvl2-PDZ exhibited clear cholesterol dependence in membrane binding ( Fig. 1a ), and bound radiolabelled cholesterol with 1:1 stoichiometry ( Supplementary Fig. 3A ). Also, it showed lower binding when cholesterol was replaced by its structural derivatives, including 5α,6β-dihydroxycholestanol, in the vesicles ( Supplementary Fig. 2B ). All these results support the notion that Dvl2-PDZ specifically interacts with cholesterol. The full-length Dvl2 also bound to cholesterol-containing membranes with high affinity and specificity, and truncation of the PDZ domain from Dvl2 abrogated its cholesterol binding ( Table 1 ), showing that Dvl2 is a cholesterol-binding protein and that the PDZ domain is fully responsible for its cholesterol binding. Table 1 Membrane affinity of Dvls, Dvl-PDZ domains and their mutants. Full size table Figure 1: Cholesterol binding of Dvl2-PDZ domain. ( a ) Cholesterol dependence of membrane binding of Dvl2-PDZ. Binding of the PDZ domain to POPC/POPS/cholesterol (80− x :20: x , x =0–40 mol%) vesicles was measured by SPR analysis. Notice that Dvl2-PDZ has significant binding to POPC/POPS (80:20) vesicles and thus the net affinity for cholesterol should be estimated by subtracting the sensorgram for POPC/POPS (80:20) vesicles from that of particular vesicles. Equilibrium SPR measurements were performed in 20 mM Tris-HCl, pH 7.4, containing 0.16 M KCl. POPC vesicles to which Dvl2-PDZ has no detectable affinity were used for the control surface. ( b ) A model structure of the Dvl2-PDZ–cholesterol–peptide ternary complex was obtained by docking cholesterol and the C-terminal Fz7 peptide to Dvl2-PDZ (PDB ID: 2REY). Cholesterol (with its hydrophobic tail pointing upwards) and the bound peptide are shown in space-filling and stick representations, respectively. Putative cholesterol-binding residues, F227 and M300, are shown in stick representation and labelled. They are predicted to partially penetrate the membrane and make contact with the hydrophobic A and B rings of cholesterol. The structure on the left panel is shown in a putative membrane-binding orientation with the dotted line indicating the membrane surface. The same model structure is also shown in a different orientation with the top surface facing the membrane (right panel). Notice that the putative lipid-binding sites are topologically distinct from the peptide-binding pocket. The model was built in the absence of the lipid bilayer and the protein may undergo further conformational changes when it binds the membrane. Full size image Dvl-PDZ domain binds a lipid and a protein simultaneously Specific cholesterol biding of Dvl2-PDZ was unexpected because it bears no homology to any cholesterol-binding proteins and lacks any known cholesterol-binding motif, such as the cholesterol recognition amino-acid consensus motif [34] or cholesterol consensus motif [35] . We thus searched for its potential membrane-binding surface according to our bioinformatics algorithms [27] , [36] . Screening of residues in the putative membrane-binding site of Dvl2-PDZ by alanine-scanning mutagenesis identified Phe-277 and Met-300 as potential binding residues for cholesterol. Detailed SPR analysis showed that mutations of Phe-277 and Met-300, either individually or in combination, with Ala caused up to a 10-fold reduction in its affinity for the PM-mimetic vesicles but exerted little effect if cholesterol was removed from the vesicles ( Table 1 ). Also, the F277A/M300A mutant (FM/A hereafter) showed markedly reduced affinity for radiolabelled cholesterol ( Supplementary Fig. 3A ) and negligible cholesterol-dependent vesicle binding ( Supplementary Fig. 3B ). Molecular modelling suggests that Phe-277 and Met-300 interact with A and B rings (that is, rings close to the hydroxyl group) of cholesterol ( Fig. 1b ). Phe-277 and Met-300 are conserved in Dvl domains, including all human Dvls and Xenopus and rat Dvl2 (see Supplementary Fig. 4 ). Collectively, these data suggest that Phe-277 and Met-300 of Dvl2 are involved in specific cholesterol binding. Molecular modelling also suggests that Dvl2-PDZ can bind cholesterol and a peptide derived from its interaction partner, Frizzled7 (Fz7) [17] , simultaneously ( Fig. 1b ) because of topological separation of two binding sites. Orthogonality of lipid and peptide binding was supported by the finding that the FM/A mutation had a negligible effect on binding of Dvl2-PDZ ( Supplementary Fig. 5A ) or the intact Dvl2 ( Supplementary Fig. 5C ) to the Fz7 peptide. Furthermore, the Fz7 peptide showed little effect on the binding of Dvl2-PDZ to PM-mimetic vesicles ( Supplementary Fig. 5B ) and vice versa ( Supplementary Fig. 5A ). Effect of Dvl-PDZ-cholesterol binding on Wnt signalling It has been reported that canonical Wnt signalling involves the binding of Dvl to the Fz–Wnt–LRP5/6 receptor complex at the PM [37] , initial phosphorylation of LRP6 by Axin–glycogen synthase kinase (GSK)3 recruited from the β-catenin destruction complex, the aggregation of the receptor complex at or beneath the PM [16] , leading to multi-site phosphorylation of LRP5/6 (ref. 38 ), and sequestration of the Axin–GSK3 complex from the β-catenin destruction complex [37] , [39] , [40] or saturation of the destruction complex [6] , [41] . The mechanisms of diverse non-canonical Wnt signalling pathways are not well understood; however, the common denominator of these pathways is the formation of the Wnt–Fz–Dvl complex [42] . We investigated the possibility that cholesterol could selectively activate canonical or non-canonical Wnt signalling by specifically facilitating key steps of each Wnt signalling pathway. Since the Dvl–Fz–Wnt interaction is involved in both canonical and non-canonical Wnt signalling, we first explored the possibility that cholesterol may differentially regulate the interaction during canonical and non-canonical Wnt signalling by single-molecule tracking analysis. This imaging method by total internal reflection fluorescence microscopy allows sensitive and accurate detection of dynamic, transient interactions among signalling proteins at the PM that may not be detected by confocal imaging or biochemical assays [28] , [43] . The analysis of the membrane residence time of the enhanced green fluorescence protein (EGFP)-tagged Dvl2 wild-type (WT) and FM/A mutant on the PM of HeLa cells showed that Dvl2 WT had much longer PM residence time than FM/A with or without Wnt ( Supplementary Fig. 6 ). This is consistent with higher PM affinity of the WT than FM/A (see Table 1 ). We then determined the co-localization time for EGFP-tagged Dvl2 (WT or FM/A) and Halo-tetramethylrhodamine (TMR)-labelled Fz7 by simultaneous tracking of the two molecules [28] , [43] . The data analysis revealed that a canonical Wnt ligand, Wnt3a, markedly increased the population of Dvl2 WT co-localized with Fz7 for >0.1 s in the PM ( Fig. 2a,b ; Supplementary Movies 1–4 ). Wnt3a also induced the aggregation of Fz7 in the presence of Dvl2 WT ( Supplementary Fig. 7 ). However, Wnt3a had no effect on the co-localization of Dvl2 FM/A with Fz7. Dvl2 FM/A molecules comigrating with Fz7 for >0.1 s were undetectable with or without Wnt3a. Also, when cholesterol in the PM of HeLa cells was depleted by methyl-β-cyclodextrin (MβCD), Wnt3a did not appreciably promote the Dvl2–Fz7 co-localization ( Fig. 3a ). Essentially the same patterns were seen in >50 different HeLa cells in each case. Also, similar patterns were observed in HEK293 cells. Since Dvl2 WT and FM/A have essentially the same chemical affinity for Fz7 (see Supplementary Fig. 5A ), these striking differences suggest that cholesterol-binding activity of Dvl2 is important for the formation and aggregation of the Dvl–Fz–Wnt complex in canonical Wnt signalling. In contrast to Wnt3a, a non-canonical Wnt, Wnt5a (or Wnt11), had little effect on co-localization of Dvl2 WT with Fz7 ( Fig. 2b ), although Wnt5a-mediated signalling should also involve the Fz7–Dvl2 interaction. Wnt5a considerably increased the short-term co-localization of Dvl2 FM/A with Fz7 (that is, 45 (mean)±10 (s.d.) to 70±10 molecules with 0.1 s co-localization) but the total number of co-localized Dvl2 FM/A–Fz7 molecules was negligible compared with the number of co-localized Dvl2 WT–Fz7 molecules under the same conditions. Taken together, these results indicate that cholesterol-binding activity of Dvl2 is important for facilitating the Dvl2–Fz7 interaction primarily in canonical Wnt signalling, which in turn suggests that cholesterol selectively activates canonical Wnt signalling through specific interaction with Dvl2-PDZ. 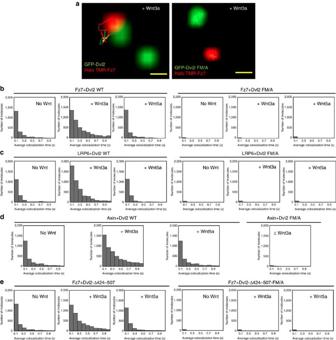Figure 2: Single-molecule tracking of Dvl and other members of the canonical Wnt signalling complex. (a) A representative pair of EGFP-tagged Dvl2 (green circles) and Halo-TMR-labelled Fz7 (red circles) in a HeLa cell is shown. The left panel is for Dvl2 WT and the right panel for FM/A. Many Dvl2 WT molecules show dynamic co-localization with Fz7 in the presence of Wnt3a (>5 min after Wnt3a stimulation), whereas most of FM/A molecules exhibit separate localization with Fz7 (see alsoSupplementary Movies 2 and 4). Green and red dots indicate individual Dvl2 and Fz7 molecules, respectively, and lines are their trajectories. Yellow scale bars indicate 0.5 μm. (b) Distribution of co-localization time of Halo-TMR-Fz7 with EGFP–Dvl2 WT or FM/A. The number of Fz7 molecules spending a given co-localzation time with Dvl2 WT on the PM of HeLa cells is displayed. Notice that Wnt3a markedly enhanced the population of Fz7 molecules co-localized with Dvl2 WT for >100 ms. In contrast, no Fz7 molecule was found to co-localized with the Dvl2 FM/A mutant for >100 ms with or without Wnt3a (see alsoSupplementary Movies 1–4). Wnt5a had no effect on Dvl2 WT or FM/A. The same size of PM surface was analysed for each histogram. (c) Distribution of co-localization time of EGFP–LRP6 with Halo-TMR-Dvl2 WT or FM/A. Wnt3a drastically enhanced the co-localization of Dvl2 WT (not FM/A) and LRP6, whereas Wnt5a had no effect on Dvl2 WT or FM/A. (d) Distribution of co-localization time of EGFP–Axin with Halo-TMR-Dvl2 WT or FM/A. Wnt3a treatment significantly increased the population of co-localized Dvl2 WT–Axin pairs while having no effect on Dvl2 FM/A–Axin co-localization. Wnt5a showed no detectable effect. (e) Distribution of co-localization time of Halo-TMR-Fz7 with EGFP–Dvl2-Δ424-507(or Δ424-507-FM/A). The two truncation mutants behaved essentially the same as their non-truncated counterparts shown inFig. 2b. Wnt3a or Wnt5a (50 ng ml−1) was used in all experiments. Figure 2: Single-molecule tracking of Dvl and other members of the canonical Wnt signalling complex. ( a ) A representative pair of EGFP-tagged Dvl2 (green circles) and Halo-TMR-labelled Fz7 (red circles) in a HeLa cell is shown. The left panel is for Dvl2 WT and the right panel for FM/A. Many Dvl2 WT molecules show dynamic co-localization with Fz7 in the presence of Wnt3a (>5 min after Wnt3a stimulation), whereas most of FM/A molecules exhibit separate localization with Fz7 (see also Supplementary Movies 2 and 4 ). Green and red dots indicate individual Dvl2 and Fz7 molecules, respectively, and lines are their trajectories. Yellow scale bars indicate 0.5 μm. ( b ) Distribution of co-localization time of Halo-TMR-Fz7 with EGFP–Dvl2 WT or FM/A. The number of Fz7 molecules spending a given co-localzation time with Dvl2 WT on the PM of HeLa cells is displayed. Notice that Wnt3a markedly enhanced the population of Fz7 molecules co-localized with Dvl2 WT for >100 ms. In contrast, no Fz7 molecule was found to co-localized with the Dvl2 FM/A mutant for >100 ms with or without Wnt3a (see also Supplementary Movies 1–4 ). Wnt5a had no effect on Dvl2 WT or FM/A. The same size of PM surface was analysed for each histogram. ( c ) Distribution of co-localization time of EGFP–LRP6 with Halo-TMR-Dvl2 WT or FM/A. Wnt3a drastically enhanced the co-localization of Dvl2 WT (not FM/A) and LRP6, whereas Wnt5a had no effect on Dvl2 WT or FM/A. ( d ) Distribution of co-localization time of EGFP–Axin with Halo-TMR-Dvl2 WT or FM/A. Wnt3a treatment significantly increased the population of co-localized Dvl2 WT–Axin pairs while having no effect on Dvl2 FM/A–Axin co-localization. Wnt5a showed no detectable effect. ( e ) Distribution of co-localization time of Halo-TMR-Fz7 with EGFP–Dvl2-Δ 424-507 (or Δ 424-507 -FM/A). The two truncation mutants behaved essentially the same as their non-truncated counterparts shown in Fig. 2b . Wnt3a or Wnt5a (50 ng ml −1 ) was used in all experiments. 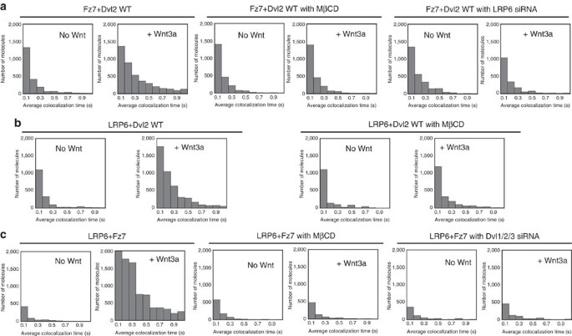Figure 3: Effects of cholesterol depletion and protein knockdown on interactions among Wnt signalling proteins in HeLa cells. (a) Effects of cholesterol depletion by methyl-β-cyclodextrin (MβCD) and LRP6 knockdown on Dvl2–Fz7 co-localization before and 10 min after stimulation by Wnt3a. (b) Effect of cholesterol depletion by MβCD on Dvl2–LRP6 co-localization before and 10 min after stimulation by Wnt3a. (c) Effects of cholesterol depletion by MβCD and Dvl1/2/3 triple knockdown on Dvl2–Fz7 co-localization before and 10 min after stimulation by Wnt3a. Protein co-localization was determined by single-molecule imaging as described forFig. 2. Wnt3a (50 ng ml−1) was used for all experiments. Cholesterol depletion was achieved by incubating cells with 1 mM MβCD in Dulbecco’s modified Eagle’s medium for 1 h at 37 °C. Short interfering RNA (siRNA) (50 nM) was used for each knockdown experiment. Full size image Figure 3: Effects of cholesterol depletion and protein knockdown on interactions among Wnt signalling proteins in HeLa cells. ( a ) Effects of cholesterol depletion by methyl-β-cyclodextrin (MβCD) and LRP6 knockdown on Dvl2–Fz7 co-localization before and 10 min after stimulation by Wnt3a. ( b ) Effect of cholesterol depletion by MβCD on Dvl2–LRP6 co-localization before and 10 min after stimulation by Wnt3a. ( c ) Effects of cholesterol depletion by MβCD and Dvl1/2/3 triple knockdown on Dvl2–Fz7 co-localization before and 10 min after stimulation by Wnt3a. Protein co-localization was determined by single-molecule imaging as described for Fig. 2 . Wnt3a (50 ng ml −1 ) was used for all experiments. Cholesterol depletion was achieved by incubating cells with 1 mM MβCD in Dulbecco’s modified Eagle’s medium for 1 h at 37 °C. Short interfering RNA (siRNA) (50 nM) was used for each knockdown experiment. Full size image To further test this hypothesis, we measured the effect of cholesterol on the Dvl2–LRP6 and Dvl2–Axin interactions that are involved only in canonical Wnt signalling. As shown in Fig. 2c , Wnt3a greatly enhanced the co-localization of Dvl2 WT and LRP6, but not that of Dvl2 FM/A and LRP6. Also, cholesterol depletion by MβCD abrogated the effect of Wnt3a on the Dvl2–LRP6 co-localization ( Fig. 3b ). In contrast to Wnt3a, Wnt5a did not affect the co-localization of Dvl2 WT (or FM/A) and LRP6. Similarly, treatment of HeLa cells expressing EGFP-tagged Axin and Halo-TMR-labelled Dvl2 WT with Wnt3a greatly increased the PM residence time of Axin ( Supplementary Fig. 8A ) and the population of the Dvl2 WT–Axin pairs with longer co-localization time at the PM ( Fig. 2d ). However, Wnt3a did not affect the co-localization of Axin with Dvl FM/A. Furthermore, Wnt5a affected neither PM localization of Axin nor its co-localization with Dvl2 at the PM ( Fig. 2d ). Since the Dvl2-PDZ is not directly involved in Axin–Dvl2 binding [5] , Dvl2 WT and FM/A should have the same chemical affinity for Axin. Thus, differential Wnt3a-induced Axin co-localization of Dvl2 WT and FM/A underscores the importance of cholesterol-binding activity of Dvl2-PDZ in mediating optimal interaction among canonical Wnt signalling proteins. To provide further evidence for this notion, we performed two additional experiments. We first monitored by single-molecule imaging the co-localization of two co-receptors of canonical Wnt signalling, Fz7 and LRP6, in HeLa cells under different conditions. Wnt3a markedly enhanced the dynamic co-localization of Fz7 and LRP6; however, cholesterol depletion by MβCD or suppression of Dvl expression by Dvl1/2/3 triple knockdown virtually abolished the Wnt3a-induced co-localization of Fz7 and LRP6 ( Fig. 3c ). We also performed co-immunoprecipitation in HEK293T cells expressing Myc-LRP6, GFP-XDvl2 (WT or FM/A) and HA-Axin. Results showed that Axin could interact with LRP6 upon Wnt3a activation only when XDvl2 WT (that is, not XDvl2 FM/A) was co-expressed ( Supplementary Fig. 9 ). Collectively, these results support the notion that cholesterol binding of Dvl2 is essential for optimal and synergistic interactions among canonical Wnt signalling proteins. We then measured how differently cholesterol binding of Dvl2 affects non-canonical Wnt signalling. Although various membrane co-receptors, including Ror [44] , [45] and Ryk [46] , [47] , and downstream effectors have been reported for different non-canonical Wnt signalling pathways, non-canonical Wnt signalling pathways do not have well-established, universal Wnt co-receptors and downstream effectors [2] , [4] , [5] . We therefore measured the interaction of Dvl2 (WT or FM/A) with Daam1 that has been reported to be a key downstream effector protein for the Wnt/PCP signalling pathway [48] , [49] . As expected from its role as a canonical Wnt, Wnt3a had little effect on the membrane residence time of EGFP-tagged Daam1 ( Supplementary Fig. 8B ) or its interaction with Halo-TMR-labelled Dvl2 WT ( Supplementary Fig. 8C ). Under the same conditions, Wnt5a (or Wnt11) modestly enhanced the PM residence time of Damm1, but had essentially no effect on its co-localization with Dvl2 WT. Consequently, Dvl2 WT and FM/A, despite having distinctively different cholesterol-binding activity, behaved similarly in terms of Wnt5a-induced co-localization with Daam1. These results suggest that Daam1 does not form a stable complex with Dvl2 on the PM during non-canonical Wnt/PCP signalling. Taken together, these results are consistent with the notion that cholesterol binding of Dvl2 plays much more important roles in canonical Wnt signalling than in non-canonical Wnt signalling. Last, we assessed the potential contribution from other parts of the Dvl2 molecule to its binding to Fz7 based on the report that the DEP domain and the C-terminal end of Dvl could tightly bind the intracellular loops of Fz5 (ref. 19 ). We measured the effect of deleting the DEP domain and the C-terminal end (Δ 424-507 ) of Dvl2 on dynamic Fz7–Dvl2 co-localization in HeLa cells. As shown in Fig. 2e , the Dvl2-Δ 424-507 mutant behaved essentially the same as the WT in terms of Wnt3a-induced co-localization with Fz7. Also, Dvl2-Δ 424-507 -FM/A and FM/A had similar properties. In conjunction with our in vitro data showing that PDZ deletion abrogates the cholesterol binding of Dvl2, these results confirm that the PDZ domain is primarily responsible for cholesterol-dependent Fz7 binding of Dvl2. Local cholesterol levels and canonical Wnt signalling Our results clearly show that cholesterol selectively activates canonical over non-canonical Wnt signalling by specifically promoting interaction of Dvl with PM and other canonical Wnt signalling proteins, most notably LRP6 and Axin. Given that both canonical and non-canonical Wnt signalling involves PM recruitment of Dvl and its interaction with the Wnt-activated Fz, a question arises as to how canonical Wnt proteins can effectively trigger the cholesterol-dependent PM and Fz binding of Dvl2, whereas non-canonical Wnt proteins cannot. One possible explanation is that canonical Wnt proteins specifically enhance the local cholesterol concentration near the Wnt signalling complex. To test this notion, we measured the change in the local cholesterol concentration in the vicinity of Fz7 in response to activation by Wnt3a and Wnt5a. To date the exact cholesterol concentration in any cellular membrane, including PM, has not been quantified in living cells or tissues in a spatiotemporally resolved manner. As an alternative approach, we monitored the spatiotemporal relationship between cholesterol and Fz7 before and after Wnt stimulation by simultaneous single-molecule tracking, which allows accurate determination of individual molecular locations [50] , of Fz7 and a cholesterol probe. The D4 domain of perfringolysin O is known to have high cholesterol specificity, but shows relatively low affinity for cholesterol-containing vesicles [51] , [52] . We thus used the EGFP-tagged D434A mutant of the D4 domain, which has higher cholesterol affinity than the WT D4 domain [53] , as a cholesterol probe in this study. 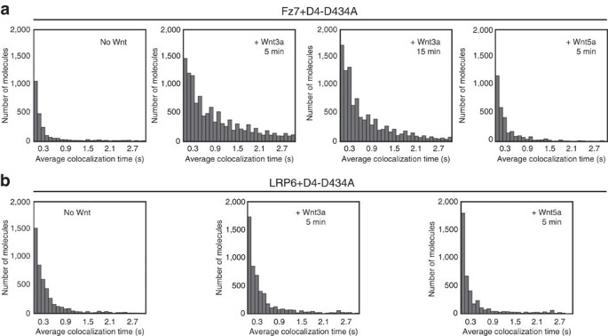Figure 4: Wnt-induced local cholesterol concentration changes estimated by a cholesterol probe. (a) Distribution of co-localization time of Halo-TMR-Fz7 with EGFP–D4-D434A before and after Wnt3a or Wnt5a treatment. Co-localization was markedly increased in response to Wnt3a stimulation and lasted for >20 min under our experimental conditions. (b) Distribution of co-localization time of Halo-TMR-D4-D434A with EGFP–LRP6 before and after Wnt3a and Wnt5a treatment. Notice that D4-D434A and EGFP–LRP6 are significantly co-localized even in the absence of Wnt3a; consequently, Wnt3a stimulation enhanced the overall co-localization only modestly. Wnt3a or Wnt5a (50 ng ml−1) was used in all experiments. Figure 4a shows that the population of the D4-D434A–EGFP co-localized with Halo-TMR-labelled Fz7 markedly increases within 5 min of Wnt3a stimulation and the phenomenon lasted for at least 20 min. Separate single-molecule analysis of D4-D434A–EGFP showed that its total PM-bound population and PM residence time remained relatively unchanged before and after Wnt3a stimulation ( Supplementary Fig. 10 ). This suggests that the increase of local cholesterol concentration surrounding Wnt3a-bound Fz7 is primarily mediated by lateral movement of cholesterol within the PM. Under the same conditions, Wnt5a stimulation caused a much lower degree of D4-D434A–Fz7 co-localization ( Fig. 4a ). These results suggest that a canonical Wnt protein (but not a non-canonical Wnt) can increase the local concentration of cholesterol in the vicinity of Fz7 at the inner leaflet of the PM. Figure 4: Wnt-induced local cholesterol concentration changes estimated by a cholesterol probe. ( a ) Distribution of co-localization time of Halo-TMR-Fz7 with EGFP–D4-D434A before and after Wnt3a or Wnt5a treatment. Co-localization was markedly increased in response to Wnt3a stimulation and lasted for >20 min under our experimental conditions. ( b ) Distribution of co-localization time of Halo-TMR-D4-D434A with EGFP–LRP6 before and after Wnt3a and Wnt5a treatment. Notice that D4-D434A and EGFP–LRP6 are significantly co-localized even in the absence of Wnt3a; consequently, Wnt3a stimulation enhanced the overall co-localization only modestly. Wnt3a or Wnt5a (50 ng ml −1 ) was used in all experiments. Full size image To investigate the mechanism underlying this new finding, we also measured the co-localization of EGFP–LRP6 with Halo-TMR-labelled D4-D434A. In contrast to Fz7, LRP6 showed a significant degree of co-localization with D4-D434A even in the absence of Wnt3a ( Fig. 4b ). As a result, the increase in co-localization of LRP6 and D4-D434A after Wnt3a stimulation was much smaller than seen with the Fz7–D4-D434A pair ( Fig. 4b ). Also, Wnt5a had no effect on LRP6–D4-D434A co-localization. It has been reported that LRP6 is located in cholesterol-rich lipid rafts and caveoli [54] , [55] , suggesting that the local cholesterol concentration around LRP6 may be higher than other locations at the PM. Our results indicate that cholesterol is indeed enriched around LRP6 molecules in the resting state, whether or not they are located in cholesterol-rich membrane domains, and that Wnt3a stimulation brings Fz7 and Dvl2 to this cholesterol-enriched microenvironment through LRP6 binding. This notion is further supported by the fact that suppression of LRP6 expression reduced the Wnt3a-induced co-localization of Fz7 and Dvl2 as much as cholesterol depletion by MβCD did (see Fig. 3a ). Cholesterol activates canonical Wnt signalling in vivo To check whether the Dvl–cholesterol interaction also selectively activates canonical Wnt signalling over non-canonical Wnt signalling under physiological conditions, we first injected into Xenopus embryos messenger RNAs (mRNAs) of either WT or FM/A mutant of Xenopus Dvl2 (XDvl2). When ventrally injected, XDvl2 FM/A was only 50% as efficient as WT in inducing the secondary axis, a readout for canonical Wnt activity ( Fig. 5a,b ). Intriguingly, XDvl2 FM/A caused more pronounced convergent extension (CE) defective phenotypes ( Supplementary Fig. 11A,B ) and Wnt/PCP-downstream JNK phosphorylation ( Supplementary Fig. 11C ) than XDvl2 WT, indicating that the mutant activated non-canonical Wnt signalling even more proficiently than WT. This result is consistent with the notion that cholesterol binding of Dvl is not involved in activation of non-canonical Wnt signalling leading to CE and PCP pathways. Presumably, exogenous XDvl2 FM/A is more active than exogenous XDvl2 WT in these non-canonical Wnt signalling assays because the former is mostly dedicated to non-canonical Wnt signalling, whereas the latter partitions between canonical and non-canonical Wnt signalling. 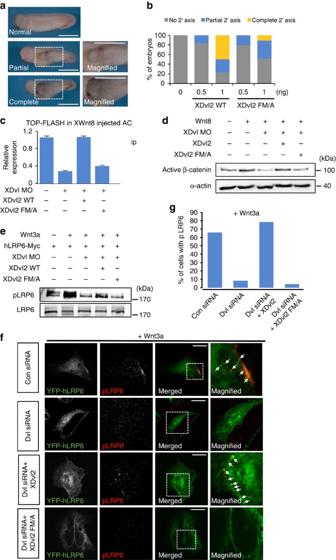Figure 5: Cholesterol binding of Dvl is required for canonical Wnt signalling under physiological conditions. (a) Induction of the secondary axis by exogenous addition of XDvl2. The partial axis was characterized by the axial structure without the head structure, including eyes and cement glands. The complete axis has the axial structure along with the head structure. Scale bar, 1 mm. (b) Quantification ofFig. 5a. (c) The TOP-flash activity was measured inXenopusAC explants. XWnt8 mRNAs were injected with indicated XDvl2 mRNAs and XDvl Morpholinos (MO). At stage 10, ACs were dissected and analysed. Error bars indicate s.d. from three independent analyses. (d) The western blot analysis of activated (dephosphorylated) β-catenin levels. α-Actin was used as a loading control. (e) Western blot data showing the degree of LRP6 phosphorylation.Xenopusembryos were injected with indicated mRNAs, including human Myc-tagged LRP6 (hLRP6-Myc), and AC tissue explants were analysed at stage 10.5. Only exogenous Dvl2 WT could rescue Dvl MO-mediated inhibition of LRP6 phosphorylation inXenopusAC tissues. hLRP6-Myc was immunoprecipitated by the c-Myc antibody and phosphorylated LRP6 (pLRP6) was detected with the antibody against Sp1490. (f) Confocal images of HeLa cells showing the location and degree of LRP6 phosphorylation. The Wnt3a-mediated co-localization (see white arrows) of GFP-human LRP6 (hLRP6) (green) and phosphorylated LRP6 at Ser1490 (pLRP6: red) was clearly seen at the PM and endosomes in control cells (Con short interfering RNA (siRNA): first row). Dvl siRNA (second row) abrogated the co-localization of hLRP6 and pLRP6, which was significantly rescued by XDvl2 (third row), but not by XDvl2 FM/A (bottom row). Scale bar, 20 μm. (g) Quantification ofFig. 5f. Figure 5: Cholesterol binding of Dvl is required for canonical Wnt signalling under physiological conditions. ( a ) Induction of the secondary axis by exogenous addition of XDvl2. The partial axis was characterized by the axial structure without the head structure, including eyes and cement glands. The complete axis has the axial structure along with the head structure. Scale bar, 1 mm. ( b ) Quantification of Fig. 5a . ( c ) The TOP-flash activity was measured in Xenopus AC explants. XWnt8 mRNAs were injected with indicated XDvl2 mRNAs and XDvl Morpholinos (MO). At stage 10, ACs were dissected and analysed. Error bars indicate s.d. from three independent analyses. ( d ) The western blot analysis of activated (dephosphorylated) β-catenin levels. α-Actin was used as a loading control. ( e ) Western blot data showing the degree of LRP6 phosphorylation. Xenopus embryos were injected with indicated mRNAs, including human Myc-tagged LRP6 (hLRP6-Myc), and AC tissue explants were analysed at stage 10.5. Only exogenous Dvl2 WT could rescue Dvl MO-mediated inhibition of LRP6 phosphorylation in Xenopus AC tissues. hLRP6-Myc was immunoprecipitated by the c-Myc antibody and phosphorylated LRP6 (pLRP6) was detected with the antibody against Sp1490. ( f ) Confocal images of HeLa cells showing the location and degree of LRP6 phosphorylation. The Wnt3a-mediated co-localization (see white arrows) of GFP-human LRP6 (hLRP6) (green) and phosphorylated LRP6 at Ser1490 (pLRP6: red) was clearly seen at the PM and endosomes in control cells (Con short interfering RNA (siRNA): first row). Dvl siRNA (second row) abrogated the co-localization of hLRP6 and pLRP6, which was significantly rescued by XDvl2 (third row), but not by XDvl2 FM/A (bottom row). Scale bar, 20 μm. ( g ) Quantification of Fig. 5f . Full size image To further elaborate in vivo functions of cholesterol binding of Dvl, we suppressed the level of endogenous X Dvl1/2/3 by triple knockdown, reintroduced either XDvl2 WT or FM/A and measured canonical Wnt signalling activities by various assays. First, we measured the degree of XWnt8-induced transcriptional activation ( Fig. 5c ) and active (dephosphorylated) β-catenin stabilization ( Fig. 5d ) in Xenopus animal cap (AC) cells by the TOP-flash assay and western blot analysis, respectively. In these assays, XDvl2 WT fully restored the suppressed endogenous Dvl activities, whereas XDvl2 FM/A did not. We also determined the extent of LRP6 phosphorylation at the PM and endosomes [16] by western blotting in Xenopus AC cells ( Fig. 5e ) and by confocal imaging ( Fig. 5f,g ) in HeLa cells, respectively. These measurements showed that XDvl2 WT could rescue LRP6 phosphorylation at the PM and endosomes much more efficiently than XDvl2 FM/A when endogenous XDvls or human Dvls were suppressed. Furthermore, XDvl2 WT could rescue canonical Wnt signalling in Dvl-morphant embryos in terms of early dorsal specification (Xnr3) ( Fig. 6a,b ), paraxial mesoderm induction (MyoD), anteroposterior neural patterning (forebrain (BF1) and midbrain-hindbrain boundary (En2)) and neural crest development (Twist) ( Fig. 6c,d ), whereas FM/A could not. Cholesterol dependency of the canonical Wnt signalling activities was further evidenced by the fact that the degrees of XWnt8-induced active β-catenin stabilization and LRP6 phosphorylation, respectively, in Xenopus AC cells were greatly reduced by cholesterol depletion by MβCD ( Supplementary Fig. 12A ). 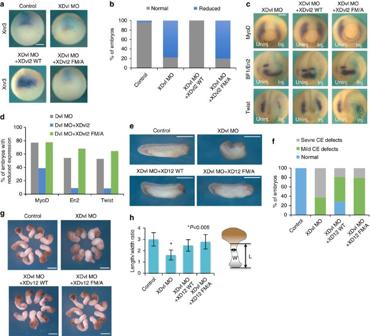Figure 6: Differential Effects of cholesterol on canonical and non-canonical Wnt signalling duringXenopusembryogenesis. (a) Xnr3 expression was analysed byin situhybridization. Embryos were injected with the indicated reagents at the dorsal side of the four-cell stage with a lineage tracer β-galactosidase mRNA and analysed at stage 10.5. Scale bar, 250 μm. (b) Quantification ofFig. 6a. (c) One side of each embryo was injected with the indicated reagents at the four-cell stage with a β-galactosidase mRNA. Expressions of MyoD at stage12, and BF1, En2 and Twist at stages 17–19 were monitored on both injected (inj.) and uninjected (uninj.) sides byin situhybridization. Scale bar, 250 μm. (d) Quantification ofFig. 6c. Percentage of embryos with reduced gene expression on the injected side was counted. (e) Reagents were introduced into the dorsal marginal region of the four-cell stage embryos and defective phenotypes were counted at tadpole stages. Severe defects were characterized by the shortened and kinked body axis, and mild defects by the slightly shortened and defective head structure. Scale bar, 1 mm. (f) Quantification ofFig. 6e. (g) DMZs were dissected at stage 10 and cultured up to stage 18. Each image was a representative of three independent experiments. Scale bar, 0.4 mm. (h) Quantification ofFig. 6g. TheYaxis indicates the length/width ratio (L/W) of each DMZ. Error bars denote s.d. Asterisk indicatesP<0.005 (determined by the two-tailedt-test) when compared with the control, (XDvl MO+XDvl2)- and (XDvl MO+XDvl2 FM/A)-injected explants, respectively. For all experiments, endogenous XDvl levels were suppressed by triple MO, and XDvl2 WT or FM/A was reintroduced to embryos. Figure 6: Differential Effects of cholesterol on canonical and non-canonical Wnt signalling during Xenopus embryogenesis. ( a ) Xnr3 expression was analysed by in situ hybridization. Embryos were injected with the indicated reagents at the dorsal side of the four-cell stage with a lineage tracer β-galactosidase mRNA and analysed at stage 10.5. Scale bar, 250 μm. ( b ) Quantification of Fig. 6a . ( c ) One side of each embryo was injected with the indicated reagents at the four-cell stage with a β-galactosidase mRNA. Expressions of MyoD at stage12, and BF1, En2 and Twist at stages 17–19 were monitored on both injected (inj.) and uninjected (uninj.) sides by in situ hybridization. Scale bar, 250 μm. ( d ) Quantification of Fig. 6c . Percentage of embryos with reduced gene expression on the injected side was counted. ( e ) Reagents were introduced into the dorsal marginal region of the four-cell stage embryos and defective phenotypes were counted at tadpole stages. Severe defects were characterized by the shortened and kinked body axis, and mild defects by the slightly shortened and defective head structure. Scale bar, 1 mm. ( f ) Quantification of Fig. 6e . ( g ) DMZs were dissected at stage 10 and cultured up to stage 18. Each image was a representative of three independent experiments. Scale bar, 0.4 mm. ( h ) Quantification of Fig. 6g . The Y axis indicates the length/width ratio (L/W) of each DMZ. Error bars denote s.d. Asterisk indicates P <0.005 (determined by the two-tailed t -test) when compared with the control, (XDvl MO+XDvl2)- and (XDvl MO+XDvl2 FM/A)-injected explants, respectively. For all experiments, endogenous XDvl levels were suppressed by triple MO, and XDvl2 WT or FM/A was reintroduced to embryos. Full size image We then measured the non-canonical Wnt signalling activities, CE-mediated elongation of embryonic body ( Fig. 6e ) and dorsal marginal zone (DMZ) explants ( Fig. 6g ) under the same conditions. Statistical analysis showed that CE defects caused by XDvl morpholinos (MO) were significantly rescued by both XDvl2 WT and XDvl2 FM/A ( Fig. 6f ), although the former was slightly more efficient than the latter. Also, the extension of the DMZ explants ( Fig. 6h ) suppressed by XDvl MO was essentially fully restored by both XDvl2 WT and XDvl2 FM/A. Furthermore, cholesterol depletion by MβCD did not affect the level of the phosphorylated JNK in dissected Xenopus DMZ tissues ( Supplementary Fig. 12B ). Collectively, these results support the notion that cholesterol binding of Dvl2 selectively activates canonical over non-canonical Wnt signalling under physiological conditions. Last, we confirmed the differential effects of cholesterol binding of Dvl2 on canonical and non-canonical Wnt signalling in HEK293FT cells. We first suppressed the expression of endogenous Dvl by short interfering RNA-mediated triple knockdown of Dvl1/2/3 and reintroduced XDvl2 WT or FM/A, and measured the canonical and non-canonical Wnt signalling activities by various assays. Both the TOP-flash assay ( Fig. 7a ) and quantification of the active β-catenin level ( Fig. 7b ) showed that Dvl2 WT could rescue the canonical Wnt signalling activities, whereas Dvl2 FM/A could not. However, both Dvl2 WT and FM/A were able to effectively rescue the non-canonical Wnt activity monitored by the level of JNK phosphorylation ( Fig. 7c ). 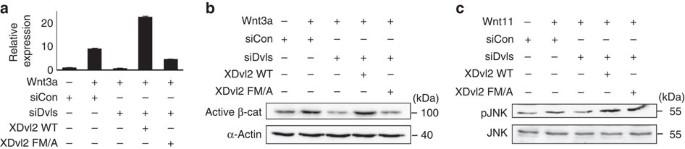Figure 7: Cholesterol binding of Dvl2 is required only for canonical Wnt signalling in culture cells. (a–c) TOP-flash activity (a), activated β-catenin level (b) and phosphorylated JNK level (c) were measured in HEK293FT cells. (a) HEK293FT cells were transfected with 50 nM of control short interfering RNA (siRNA) or Dvl1/2/3 siRNAs along with TOP-flash reporter constructs and Dvl DNAs before 24 h of Wnt3a conditioned medium stimulation. Error bars indicate s.d. from three independent analyses. (b,c) HEK293FT cells were transfected with indicated siRNAs and DNAs before 6 h of Wnt3a stimulation (b) or 1 h of Wnt11 stimulation (c). Cell lysates were harvested and analysed by western blotting with activated β-catenin (b) or phosphorylated JNK antibodies (c). Actin and JNK levels were used as loading controls. Figure 7: Cholesterol binding of Dvl2 is required only for canonical Wnt signalling in culture cells. ( a – c ) TOP-flash activity ( a ), activated β-catenin level ( b ) and phosphorylated JNK level ( c ) were measured in HEK293FT cells. ( a ) HEK293FT cells were transfected with 50 nM of control short interfering RNA (siRNA) or Dvl1/2/3 siRNAs along with TOP-flash reporter constructs and Dvl DNAs before 24 h of Wnt3a conditioned medium stimulation. Error bars indicate s.d. from three independent analyses. ( b , c ) HEK293FT cells were transfected with indicated siRNAs and DNAs before 6 h of Wnt3a stimulation ( b ) or 1 h of Wnt11 stimulation ( c ). Cell lysates were harvested and analysed by western blotting with activated β-catenin ( b ) or phosphorylated JNK antibodies ( c ). Actin and JNK levels were used as loading controls. Full size image This study shows that Dvl is a cholesterol-binding protein and that specific cholesterol binding of Dvl is important for its role in the canonical Wnt signalling pathway. Different models have been proposed for the activation of the canonical Wnt signalling pathway, but a common denominator is Dvl-mediated organization of a Wnt receptor signalling complex at the PM (and endosomes) that leads to multi-site phosphorylation of LRP5/6 and sequestration of Axin–GSK3 from the β-catenin destruction complex [2] , [4] , [5] . It was reported that direct interaction between Dvl-PDZ and Fz is relatively weak, and that other factors may be necessary for high-fidelity signal transduction between the two molecules [17] . Our results suggest that cholesterol may play such a role. Cholesterol is a major lipid component of the mammalian PM. Since cholesterol is a hydrophobic molecule with a small polar headgroup, it is located close to the hydrophobic interior of the membrane. Thus, cholesterol binding of any cytosolic protein, including Dvl, would involve its initial interaction with anionic lipids, such as PS or PtdIns(4,5)P 2 , in the PM, which is consistent with our finding (see Supplementary Fig. 2A ). This initial step is followed by partial penetration of the protein into the membrane core, which is known to enhance the membrane residence time of the protein and its sustained interaction with binding partner proteins in the membrane [28] , [31] . Indeed, our single-molecule tracking ( Fig. 2 ) shows that cholesterol binding of Dvl2 via its PDZ domain enhances its PM population, PM residence time and dynamic co-localization with Fz7 and other components of canonical Wnt signalling, including LRP6 and Axin, on the inner layer of PM in response to Wnt3a stimulation. In contrast, formation of the Wnt/PCP signalling complex containing Daam1 is independent of the cholesterol-binding activity of Dvl2 under the same conditions. Dvl is a key factor in both canonical and non-canonical Wnt signalling pathways, but the mechanisms by which it differentially triggers these pathways are poorly understood [5] . On the basis of our results, we propose a model ( Fig. 8 ) in which cholesterol binding of Dvl is essential for its scaffolding function in canonical Wnt signalling. Our model posits that canonical Wnt ligand induces the initial formation of the Dvl–Fz–Wnt–LRP6 complex at PM, which in turns raises the local cholesterol concentration in the vicinity of the complex, as these molecules are recruited to the cholesterol-enriched microenvironment of LRP6. This local cholesterol enrichment then allows tighter binding of Dvl to the membrane and other protein molecules in the complex, which promotes LRP6 phosphorylation, aggregation of the complex and recruitment of other proteins, including Axin and GSK3, to the complex. Our results suggest that for non-canonical Wnt signalling, most notably Wnt/PCP signalling, cholesterol is dispensable for the overall scaffolding function of Dvl, presumably because sustained PM residence of Dvl and the formation of a stable signalling complex at the PM is not necessary for this pathway. Our results also show that the DEP domain and the C-terminal end of Dvl2 are not involved in cholesterol-induced membrane and protein binding of Dvl2 in canonical Wnt signalling. It is possible, however, that their interaction with anionic lipids and Fz may play a more predominant role in non-canonical Wnt signalling [56] . 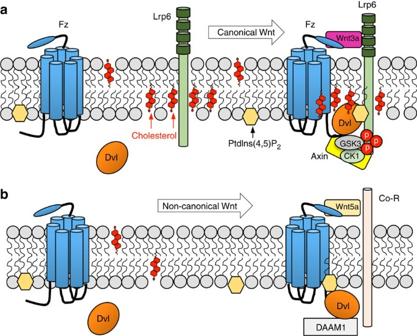Figure 8: A model for cholesterol-mediated canonical Wnt signalling-specific functions of Dvl. (a) Binding of a canonical Wnt to the Fz7 and LRP6 receptors induces the local enrichment of cholesterol in the vicinity of the activated receptor complex by bringing Fz7 closer to LRP6 in a cholesterol-enriched microenvironment. This concomitantly recruits Dvl to the complex through its coincident recognition of Fz7 and cholesterol (and an anionic lipid, such as PtdIns(4,5)P2) by its PDZ domain. Cholesterol binding of Dvl ensures the canonical Wnt signalling-specific scaffolding function of Dvl by allowing sustained interaction of Dvl with Fz7 and other proteins involved in canonical Wnt signalling, including Axin and GSK3, and thereby facilitating LRP6 phosphorylation. The canonical Wnt signalling complex containing phosphorylated LRP6 can also be endocytosed to continue signalling activities intracellularly. (b) By contrast, cholesterol binding of Dvl is not required for non-canonical Wnt signalling (for example, Wnt/PCP signalling), because its scaffolding activity for proteins involved in these pathways (for example, Daam1) does not seem to depend on its sustained PM localization. Co-R indicates a potential co-receptor for non-canonical Wnt signalling. Other putative steps of canonical Wnt signalling, including receptor complex aggregation, local PtdIns(4,5)P2enrichment6,37,41, and the downstream Wnt signalling events are omitted here for simplicity. Figure 8: A model for cholesterol-mediated canonical Wnt signalling-specific functions of Dvl. ( a ) Binding of a canonical Wnt to the Fz7 and LRP6 receptors induces the local enrichment of cholesterol in the vicinity of the activated receptor complex by bringing Fz7 closer to LRP6 in a cholesterol-enriched microenvironment. This concomitantly recruits Dvl to the complex through its coincident recognition of Fz7 and cholesterol (and an anionic lipid, such as PtdIns(4,5)P 2 ) by its PDZ domain. Cholesterol binding of Dvl ensures the canonical Wnt signalling-specific scaffolding function of Dvl by allowing sustained interaction of Dvl with Fz7 and other proteins involved in canonical Wnt signalling, including Axin and GSK3, and thereby facilitating LRP6 phosphorylation. The canonical Wnt signalling complex containing phosphorylated LRP6 can also be endocytosed to continue signalling activities intracellularly. ( b ) By contrast, cholesterol binding of Dvl is not required for non-canonical Wnt signalling (for example, Wnt/PCP signalling), because its scaffolding activity for proteins involved in these pathways (for example, Daam1) does not seem to depend on its sustained PM localization. Co-R indicates a potential co-receptor for non-canonical Wnt signalling. Other putative steps of canonical Wnt signalling, including receptor complex aggregation, local PtdIns(4,5)P 2 enrichment [6] , [37] , [41] , and the downstream Wnt signalling events are omitted here for simplicity. Full size image Controlling a balance between canonical and non-canonical Wnt signalling activities is known to be important for physiological regulation [57] , as evidenced by hematopoietic stem cell aging caused by a canonical to non-canonical Wnt signalling switch [58] . However, the mechanism underlying this control is not fully understood because the specificity of Wnt proteins for canonical versus non-canonical Wnt signalling may vary depending on the biological context [57] . Our results suggest a potential link between intracellular cholesterol levels at the PM and the balance between canonical and non-canonical Wnt signalling activities. It has been generally believed that cellular cholesterol levels are tightly regulated by the cholesterol-sensing system in the endoplasmic reticulum [59] , [60] . However, abnormal cholesterol levels have been implicated in several diseases, including cardiovascular disease, Niemman-Pick type C disease and Alzheimer’s disease, among others [20] , [61] . It has been also shown that exposure to atherogenic lipoproteins and hypercholesterolaemia in vivo results in a two- to threefold increase in overall cholesterol level in several cell types [62] , [63] . Although it is generally believed that cholesterol levels at the PM will vary according to these changes in cellular cholesterol levels, the actual cholesterol levels at different cellular locations, including two leaflets of mammalian PM, have not been quantitatively determined under physiological conditions. High spatial resolution of single-molecule imaging allowed for two novel findings: a significant local enrichment of cholesterol surrounding LRP6 in the inner leaflet of PM in the resting state and a large degree of increase in the local cholesterol concentration in the vicinity of the Wnt3a-activated Fz7 receptor. Most importantly, these results support Wnt3a-induced local cholesterol enrichment surrounding the canonical Wnt signalling complex, resulting in selective activation of canonical Wnt signalling over non-canonical Wnt signalling (see above and Fig. 8 ). It has been reported that LRP6 is localized in cholesterol-rich lipid rafts [54] , [55] . It should be noted that the local cholesterol enrichment in the vicinity of LRP6 and Wnt3a–Fz7–LRP6 observed in our study does not necessarily mean that they are located in cholesterol-rich membrane microdomains, such as lipid rafts, containing other lipid and protein components. Cholesterol binding of Dvl2-PDZ follows a stoichiometric Langmuir-type pattern (see Fig. 1a ; Supplementary Fig. 1 ). This indicates that the activity of Dvl would respond spontaneously to the change in local cholesterol concentration and would not depend on the formation of cholesterol-rich microdomains. In other words, cholesterol would serve as a genuine regulatory lipid that directly and specifically controls the canonical Wnt signalling activities of Dvl without having to form cholesterol-rich microdomains, if the local cholesterol concentration varies in response to specific stimuli. Undoubtedly, further studies are necessary to accurately quantify the cholesterol concentration in a spatiotemporally resolved manner [64] and to elucidate the mechanism underlying the local cholesterol enrichment. Nevertheless, our present study provides new mechanistic insight into the differential regulation of canonical and non-canonical Wnt signalling pathways, and suggests a potential link between cellular cholesterol levels and the balance between canonical and non-canonical Wnt signalling activities. It also raises the possibility of specific pharmacological inhibition of canonical Wnt signalling through modulation of the Dvl–cholesterol interaction. Materials The complementary DNAs (cDNAs) for the full-length human Dvl and their PDZ domains were subcloned into pET-30a(+) (Invitrogen) or pEGFPC1 (BD Clonetech) vectors, respectively. The cDNA for the full-length XDvl2 was modified at its 5′ end to make it insensitive to the XDvl MO (Geen-Tools). MO sequences used were 5′-GGTAGATGATTTTGGTCTCAGCCAT-3′ ( X Dvl1), 5′-TCACTTTAGTCTCCGCCATTCTGCG-3′ ( X Dvl2) and 5′-GGTAGATGACCTTGGTCTCCCCCAT-3′ ( X Dvl3). siRNAs (ST Pharm Co.) used in this study were 5′-CACGACCAAGGCCTATACA-3′ (human Dvl1), 5′-TCCACAATGTCTCTCAATA-3′ (human Dvl2), 5′-TAAACGAGATCAACTTTGA-3′ (human Dvl3) and 5′-ACATTGTTCTGCAGTTAGC-3′ (human LRP6). GFP-XDvl2 (ref. 46 ), myc-XFz7 (ref. 65 ), myc-XWnt8 and myc-XWnt11 plasmids [46] were prepared as described previously. The cDNA for the PFO D4 domain was a generous gift from Dr Alejandro P. Heuck of University of Massachusetts. Mutagenesis was performed using the QuickChange kit (Stratagene) or by PCR using Pfu polymerase. All constructs were confirmed by DNA sequencing. Antibodies against actin, HA, GFP and c-Myc were from Santa Cruz. Antibodies against JNK, phospho-JNK, LRP6 (C5C7), Dvl2 and phospho-LRP6 (Ser1490) were from Cell Signaling. The activated β-catenin antibody and the anti-glyceraldehyde-3-phosphate dehydrogenase antibody were from Millipore, and Alexa Fluor 594 goat anti-rabbit IgG from Life Technologies. HeLa, HEK293 and HEK293T cells were from ATCC and HEK293FT from Life Technologies. Protein expression and purification All Dvl constructs containing a C-terminal His 6 tag were transformed into BL21(DE3)pLys (Novagen) cells for protein expression. Expressed proteins were loaded onto the Ni-NTA (Qiagen) agarose resin and eluted with 50 mM Na 2 HPO 4 , pH 8.0, 300 mM NaCl containing 50–150 mM imidazole. Fractions were then pooled and the further purified on a Q-Sepharose ion-exchange column. Protein concentration was then determined by the bicinchoninic acid method (Pierce). The proteins were stored at −80 °C for further study. Lipid vesicle preparation PM-mimetic vesicles were prepared by mixing 1-palmitoyl-2-oleoyl- sn -glycero-3-phosphocholine, 1-palmitoyl-2-oleoyl- sn -glycero-3-phosphoethanolamine, 1-palmitoyl-2-oleoyl- sn -glycero-3-phosphoserine, cholesterol, 1-palmitoyl-2-oleoyl- sn -glycero-3-phosphoinositol and 1,2-dipalmitoyl derivatives of phosphatidylinositol-(4,5)-bisphosphate (PtdIns(4,5)P 2 ) in a molar ratio of 12:35:22:22:8:1. Large unilamellar vesicles with 100-nm diameter were prepared with a Liposofast (Avestin) microextruder using a 100-nm polycarbonate filter. Lipid–protein and protein–protein binding measurements All SPR measurements were performed at 23 °C in 20 mM Tris-HCl, pH 7.4, containing 0.16 M KCl using a lipid-coated L1 chip in the BIACORE X system as described previously [66] . PM-mimetic (or other) vesicles and 1-palmitoyl-2-oleoyl- sn -glycero-3-phosphocholine vesicles were injected (5 μl min −1 ) onto the active surface and the control surface of the sensor chip, respectively, to yield the identical resonance units. Equilibrium measurements were performed at a flow rate of 5 μl min −1 to allow the resonance unit values for the association phase to reach near equilibrium ( R eq ). Each sensorgram was background-corrected by subtracting the control surface response from the active surface response. A minimum of five different protein concentrations were injected to collect a set of R eq values that were plotted against the protein concentrations ( P o ). An apparent dissociation constant ( K d ) was then determined by nonlinear least-squares analysis of the binding isotherm using the equation, R eq = R max /(1+ K d / P o ), where R max indicates the maximal R eq value. Since the concentration of lipids coated on the sensor chip cannot be accurately determined, K d is defined as P o yielding half-maximal binding with a fixed lipid concentration. Each measurement was repeated at least three times to determine average and s.d. values. For kinetic measurements, the flow rate was maintained at 20–30 μl min −1 . Binding to radiolabelled cholesterol Binding of PDZ domains to mono-dispersed 1,2- 3 H-labelled cholesterol (Perkin-Elmer) was performed in 20 mM Tris-HCl, pH 7.4, with 160 mM NaCl and 1 μM of protein. Cholesterol in ethanol was added to the protein solution to a final concentration ranging from 0 to 10 μM and the mixture was incubated at 25 °C for 1 h. A His SpinTrap column (GE Healthcare) was pre-equilibrated with 20 mM Tris-HCl pH 7.4, with 160 mM NaCl and the reaction mixture was added to the column and incubated for 5 min. The column was washed three times by 600 μl of the same buffer, and the protein was eluted using 600 μl of 20 mM Tris-HCl pH 7.4, with 160 mM NaCl and 300 mM immidazole. Eluted solution (200 μl) was taken for radioactivity measurement using the Beckman LS6500 liquid scintillation counter. PDZ–peptide-binding assay by fluorescence anisotropy A fluorescein-6-aminohexanoyl (F-Ahx)-labelled Fz7 peptide, F-Ahx-GKTLQSWRRFYH was dissolved in 20 mM Tris buffer, pH 7.9, containing 160 mM NaCl, 300 mM imidazole and 5% dimethylsulphoxide. To each well of a Corning 96 flat-bottom black polystyrol plate was added 100 μl solution containing 5 nM peptide and each PDZ domain solution (100 nM to 1 mM). After 30 min incubation, the plate was inserted into Tecan Genios Pro spectrofluorometer and the fluorescence anisotropy ( r ) was measured with excitation and emission wavelengths set at 485 and 535 nm, respectively. Since P o >> Pep o under our conditions, the K d for the PDZ domain-peptide binding was determined by the nonlinear least-squares analysis of the binding isotherm using the equation (1): where Pep bound , Pep o and P o indicate the concentration of bound peptide, total peptide and total PDZ domain, respectively, and Δr and Δr max are the anisotropy change for each P o and the maximal Δr , respectively. GST pull-down experiment Glutathione S -transferase (GST) and GST-fusion peptides (GST-GKTLQSWRRFYHRLSHSSKGETAV) were expressed in Escherichia coli BL21 (DE3)pLysS and purified. The proteins were mixed with glutathione beads in the incubation buffer (20 mM Tris-HCl, pH 7.4, 0.16 M NaCl, 1% Triton X-100) and the beads with the bound proteins were washed three times with the buffer and re-suspended in the buffer. Purified human Dvl2 proteins (0–5 μg) were incubated with 5 μg of GST and GST–Fz7 for 30 min at 4 °C. The bound proteins were collected by brief centrifugation, washed three times with the incubation buffer, extracted with the Laemmli buffer and subjected to dodecylsulphate-polyacrylamide gel electrophoresis and immunoblotting using rabbit polyclonal antibodies against Dvl2 and horseradish peroxidase-conjugated goat anti-rabbit IgG. Molecular modelling of the Dvl2-PDZ–lipid–peptide complex We first built a model of the PDZ–peptide complex using the crystal structures of the Dvl2-PDZ (PDB ID: 2REY). We searched PDB database with Ska program [67] to find a PDZ domain that is complexed with a peptide and displays a high structural similarity with each PDZ domain. Once the best match had been found for Dvl2-PDZ, the PDZ domain was substituted by the structurally superimposed Dvl2-PDZ and the peptide in the crystal structure was mutated into the sequence for the Fz7 peptide using Chimera [68] . The resulting PDZ–peptide complex was subjected to FlexPepDock, a refinement tool with high-resolution peptide docking protocol. For generation of the model of Dvl2-PDZ in complex with the peptide and cholesterol, a cholesterol molecule was docked sequentially to the Dvl2-PDZ–peptide complex using the package DOCK 6. Xenopus embryo manipulation and phenotypic analysis Xenopus eggs were obtained and fertilized as described previously [69] . Human chorionic gonadotropin was injected into a female Xenopus 12 h before collecting eggs. Xenopus eggs were obtained in 1X Marc’s Modified Ringers (MR) solution and in vitro fertilized using excised testes from a male frog. Nieuwkoop and Faber stages were considered for the developmental staging. Plasmids or mRNAs were introduced into the embryos by microinjection using a Nanoliter injector (WPI) and a Harvard injector (PLI-100). Embryos were cultured in 33% MR until stage 8 and in 10% MR thereafter. For the analysis of gastrulation-defective phenotypes, endogenous XDvl levels in embryos were suppressed by triple knockdown of Dvl1/2/3 with specific MO and/or either of XDvl2 WT and FM/A was reintroduced by injection of its mRNA into embryos, and embryos were cultured until stage 32. Phenotypes were quantified as described in the figure legends. For the analysis of DMZ elongation assay, tissues were cultured until stage 18. Luciferase assay and western blotting For Wnt reporter activity, pTopflash and pRLtk were introduced along with mRNAs and/or XDvl MO into the animal pole of two-cell stage embryos. At stage 11, embryos were harvested and luciferase activities were measured using the Dual-Luciferase Reporter Assay System (Promega). Western blot analysis of pLRP6, LRP6, active (dephosphorylated) β-catenin and actin were performed from animal cap lysates, whereas pJNK and JNK were analysed from DMZ explants using specific antibodies for individual proteins. Full scans of all western blots in the main figures are shown in Supplementary Fig. 13 . In situ hybridization DIG-labelled antisense RNA probe for each gene was hybridized and the hybridizations were detected using alkaline-phosphatase-conjugated anti-digoxigenin antibody (Roche), stained with BM purple as a substrate (Roche) and photographed. Confocal and single-molecule imaging HeLa (or HEK293) cells transiently transfected with N-terminal-EGFP-tagged Dvl2 were used for confocal imaging using a Zeiss LSM510 microscope. Simultaneous single-molecule imaging of two proteins was performed in HeLa cells using a total internal reflection fluorescence microscope custom-built on the Olympus IX71 microscope base as described previously [28] . Typically, one protein is tagged with EGFP (on either N- or C terminus) and the other by Halo (Promega), which was labelled with Halo-Tag TMR (Promega) as described [28] . For efficient expression of EGFP–LRP6, a LRP6-chaperone protein Mesd [70] was co-transfected to HeLa cells. Two DPSS laser sources (488 and 561 nm, Excelsior, Spectra-Physics) were used and the fluorescence signal from the sample was split into two channels, passed through emission filters (510BP20, Omega and D630/30, Chroma), and projected onto two Andor iXon 897 EM-CCD cameras. The images were spatially corrected following the algorithm described previously [43] . All particle tracking, data analysis and image processing were carried out with in-house programs written in MATLAB. Co-localization analysis of two molecules was performed with a fixed threshold criterion (that is, <400 nm) for co-localization [43] . How to cite this article: Sheng, R. et al. Cholesterol selectively activates canonical Wnt signalling over non-canonical Wnt signalling. Nat. Commun. 5:4393 doi: 10.1038/ncomms5393 (2014).